Long-term stable polymer solar cells with significantly reduced burn-in loss The inferior long-term stability of polymer-based solar cells needs to be overcome for their commercialization to be viable. In particular, an abrupt decrease in performance during initial device operation, the so-called ‘burn-in’ loss, has been a major contributor to the short lifetime of polymer solar cells, fundamentally impeding polymer-based photovoltaic technology. In this study, we demonstrate polymer solar cells with significantly improved lifetime, in which an initial burn-in loss is substantially reduced. By isolating trap-embedded components from pristine photoactive polymers based on the unimodality of molecular weight distributions, we are able to selectively extract a trap-free, high-molecular-weight component. The resulting polymer component exhibits enhanced power conversion efficiency and long-term stability without abrupt initial burn-in degradation. Our discovery suggests a promising possibility for commercial viability of polymer-based photovoltaics towards real solar cell applications. Polymer-based solar cells (PSCs) continue to attract considerable attention because of their unprecedented advantages as low-cost, flexible and printable photovoltaics. Recent advances in the design of new conjugated polymers and in device fabrication techniques have significantly improved the power conversion efficiency (PCE), which has ultimately exceeded ~10% in laboratory-scale PSCs [1] , [2] . In addition to a high PCE, long-term stability is another key factor for the successful commercialization of PSCs [3] . Indeed, the short lifetime of organic-based devices has been considered to be their most serious disadvantage, one that must be overcome before the commercialization of these devices. Most organic photoactive materials are vulnerable to oxidation through reactions with oxygen and/or water molecules; therefore, these materials require tight encapsulation using a heavy-duty gas barrier film [4] , [5] . To prevent photoactive polymers from oxidizing, conjugated polymers with a deep highest occupied molecular orbital (HOMO) level have been developed to reduce the susceptibility to oxidation [6] . Despite intensive efforts to prolong the device lifetime, PSC devices still suffer from unexpected device degradation, even under inert atmospheres [4] , [7] , [8] . In particular, an abrupt decrease in performance during the initial stage of device operation, the so-called ‘burn-in’ loss, has frequently been observed in most PSCs and is considered to be a major contributor to the inferior lifetimes of PSCs [8] , [9] , [10] . The origin of this ‘burn-in’ loss is not yet clear and is currently a topic of considerable debate, with potential origins including oxygen trapped within the films, the broad polydispersity of the polymer samples, and organic or inorganic impurities in the polymers (such as palladium catalysts, tin- or halogen-containing molecules, unreacted monomer moieties, cross-coupling byproducts within the polymer samples and so on) [9] , [10] , [11] , [12] , [13] , [14] . This problem has also raised a fundamental question as to whether the limited lifetime of PSCs is inherent to the photoactive polymers and fundamentally cannot be overcome. Therefore, the fabrication of PSCs without this burn-in loss remains a formidable challenge in the efforts to ensure a competitive device lifetime for polymer-based photovoltaic technology. In this study, we fabricate PSCs, expecting an extremely long-term stability in which the initial burn-in loss is significantly reduced. By dividing test-bed polymers with multi-modal molecular weight (MW) distributions into three unimodal components via gel permeation chromatography (GPC) analysis ( Fig. 1 ), we are able to isolate the high-quality high-MW component that selectively rules out the components exhibiting trap-filling behaviours. The resulting high-MW component polymer exhibits a significantly enhanced PCE and a prolonged lifetime without showing an abrupt burn-in degradation. Moreover, this component-splitting approach based on GPC analysis also explains the long-standing issue of ‘batch-to-batch’ variation that might originate from the coexistence of precipitated and dissolved fractions in the same reaction flask. 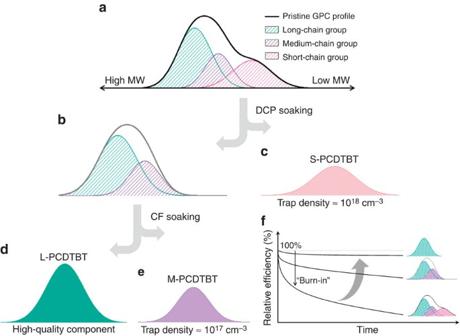Figure 1: A schematic illustration of the component-splitting approach. (a) By defining each unimodal group as a quantified unit, the componentf ractions can be individually distinguished and selectively isolated from a pristine polymer sample. The simple solvent-soaking treatment with dichloropropane (DCP) enables the extraction of (b) higher MW fractions, isolating (c) the lowest MW component. The chloroform (CF) soaking treatment makes a split between (d) high-molecular weight and (e) medium-molecular weight fractions. (f) The use of the high-quality component consequently results in the almost elimination of ‘burn-in’ for polymer solar cells. Figure 1: A schematic illustration of the component-splitting approach. ( a ) By defining each unimodal group as a quantified unit, the componentf ractions can be individually distinguished and selectively isolated from a pristine polymer sample. The simple solvent-soaking treatment with dichloropropane (DCP) enables the extraction of ( b ) higher MW fractions, isolating ( c ) the lowest MW component. The chloroform (CF) soaking treatment makes a split between ( d ) high-molecular weight and ( e ) medium-molecular weight fractions. ( f ) The use of the high-quality component consequently results in the almost elimination of ‘burn-in’ for polymer solar cells. Full size image Donor polymer material for PSC lifetime study We chose a well-known conjugated copolymer, poly[ N -9′′-hepta-decanyl-2,7-carbazole-alt-5,5-(4′,7′-di-2-thienyl-2′,1′,3′-benzothiadiazole)] (PCDTBT), as a test-bed donor material for PSC lifetime study. Because PCDTBT possesses a high oxidation potential (~5.5 eV), the oxidation of this polymer is energetically unfavourable [7] . In addition, the deep HOMO level enables a high photovoltage of up to ~1 V in photovoltaic devices [15] . Therefore, we used PCDTBT as an electron-donating polymer in combination with [6,6]-phenyl-C71-butyric acid methyl ester (PC 71 BM) as an electron-accepting material within the typical bulk heterojunction (BHJ) solar cell architecture ( Supplementary Fig. 1 ). We synthesized more than 70 batches of PCDTBT under nearly identical polymerization conditions ( Supplementary Fig. 2 ). Although we characterized the molecular and optoelectrical properties of all batch samples, we present only the most representative samples in this work (batches A to L); the characteristic features of these samples are representative of the entire range of the 70 batches. The synthesized PCDTBT samples appeared to possess nearly identical electronic structures, as implied by the absorption spectra, in which all samples exhibited common spectral features ( Supplementary Fig. 3a ). However, when we fabricated PSCs using these polymers, we observed that the current density–voltage ( J – V ) characteristics varied considerably ( Supplementary Fig. 3b ), that is, the so-called ‘batch-to-batch’ problem; although we followed nearly identical synthesis procedures, the resulting polymers exhibited different device performances for each batch ( Table 1 ). Table 1 Device and GPC parameters for PCDTBT polymer batches (A to L). Full size table Conventional assessment of polymer quality In general, a polymer material is classified by its number-averaged MW ( M n ) and polydispersity index (PDI). A higher M n and a narrower PDI typically result in high-quality electronic and optoelectronic polymer materials. This rule holds true within a certain range of values, particularly for M n ( Supplementary Fig. 3c ). For M n <20 kDa, a linear correlation between M n and PCE is clearly observed. As M n approaches ~20 kDa, the PCE value steeply increases from ~3 to ~5%. This linear dependence is attributed to oligo-to-polymeric molecular growth, as supported by the evolutions of the ultraviolet–visible absorption spectra and transition temperature ( T g ) as functions of M n ( Supplementary Fig. 3a,d ), which exhibit a trend similar to that observed in the M n -PCE correlation. In contrast, for a sufficiently high M n of over 20 kDa, where macromolecular properties become dominant, this linear correlation is no longer observed. The PCE is saturated for M n >20 kDa and fails to demonstrate any apparent correlation with M n . The PDI value is also not appropriate for classifying polymers in the macromolecular range above M n >20 kDa. For example, the highest PCE was obtained for batch A (PCE=6.16%), which possessed an even lower M n (~27 kDa) and broader PDI (~2.7) than did batch D (PCE=5.52%, M n =39 kDa, and PDI=1.9). The device parameters and the polymer-characterizing parameters of the representative batches are summarized in Table 1 . GPC analysis of PCDTBTs The M n value is typically obtained from the arithmetic mean of the integral of the MW distribution as measured via GPC analysis [16] , [17] . Thus, even though different batch samples may have almost identical M n values, those samples may exhibit considerably different MW distributions. Therefore, to search for a factor that could decisively characterize each batch, we directly examined the GPC profiles of the representative batches (A to L), as shown in Fig. 2a . Surprisingly, we found that all of the GPC profiles could be fit with a combination of three common individual distributions, each with a unimodal shape. This approach was particularly successful for the polymer batches with M n >20 kDa (that is, batches A to I), which were in the polymeric regime. However, we observed that all 70 batch samples could be perfectly described by a combination of these three components. We denote these three unimodal distributions as L-, M-, and S-PCDTBT, which represent the long-, medium- and short-chain groups of PCDTBT, respectively, and these distributions are presented in Fig. 2b for the batch I sample as an example. 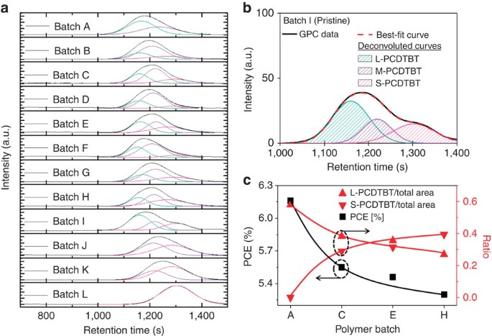Figure 2: GPC data for various batches of PCDTBT polymers. (a) GPC profiles for the as-synthesized PCDTBT polymers from batches A to L. Most of the GPC curves are composed of two or three constituent curves. The constituent curves (L-, M- and S-PCDTBTs) are represented by green, purple and red lines, respectively. (b) GPC curves that were deconvoluted through the multi-curve fitting of the pristine GPC data for the batch I sample. (c) Effects of the L- and S-PCDTBT proportions of the entire curve integrals on the device efficiency with respect to different batches (batches A, C, E, H) with similarMn(27–28 kDa). Figure 2: GPC data for various batches of PCDTBT polymers. ( a ) GPC profiles for the as-synthesized PCDTBT polymers from batches A to L. Most of the GPC curves are composed of two or three constituent curves. The constituent curves (L-, M- and S-PCDTBTs) are represented by green, purple and red lines, respectively. ( b ) GPC curves that were deconvoluted through the multi-curve fitting of the pristine GPC data for the batch I sample. ( c ) Effects of the L- and S-PCDTBT proportions of the entire curve integrals on the device efficiency with respect to different batches (batches A, C, E, H) with similar M n (27–28 kDa). Full size image We observed that the ratio of components determined the quality of each batch. When the L component (high MW) occupied more of the total area in the GPC curves, the corresponding devices exhibited higher PCEs, whereas the S component (low MW) acted as a limiting factor that decreased the device performance. This trend was apparent even among different batch samples (batches A, C, E and H) that all exhibited nearly identical M n values (27–28 kDa), as shown in Fig. 2c . A higher L-PCDTBT proportion and a lower S-PCDTBT proportion in the total GPC profile resulted in higher device efficiency, irrespective of the PDI. Therefore, we conclude that the low-MW components (M- and S-PCDTBT) in the MW distributions might be responsible for the ‘batch-to-batch’ variations in the physical properties of electronic polymers. Assuming that the multi-modal MW profiles imply the actual coexistence of individual groups in the MW distribution (L-, M- and S-PCDTBT components) that are present in a different combination for each batch, we individually extracted these three unimodal components from an arbitrarily selected batch (here batch I) using a marginal solvent-soaking technique. First we extracted the S-PCDTBT component, which primarily consisted of short chains with a relatively low MW, using dichloropropane (DCP). The second component (M-PCDTBT) was extracted from the remaining DCP-soaked polymer using chloroform cooled to low T (~5 °C). The third component (L-PCDTBT), which was expected to be composed primarily of long chains with high MW, was collected from the material remaining after the previous two extraction steps. The measured GPC profiles of these three extracted components (solid lines in Fig. 3a ) are somewhat surprising: the GPC curves are nearly coincident with the theoretically deconvoluted curves (dotted lines in Fig. 3a ). This observation clearly demonstrates that our component-splitting approach based on the unimodality of the GPC profiles is quite sound and that the theoretically deconvoluted components (L-, M- and S-PCDTBT) in fact coexisted in each batch sample. 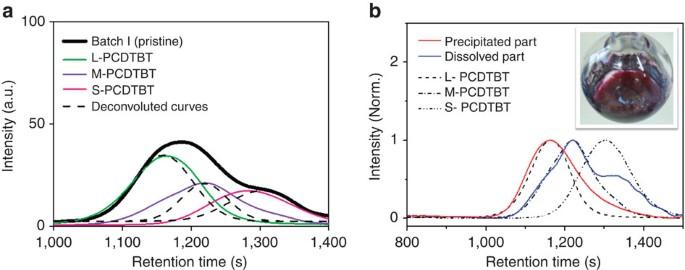Figure 3: GPC curves for split components and precipitated/dissolved fractions. (a) Polymer components (green, purple and red) extracted from the batch I sample. The dotted curves were virtually deconvoluted from the GPC data for the batch I sample. (b) The inset photograph shows the precipitated and dissolved products in a reaction flask after polymerization process. The red GPC curve is for the synthetic product of PCDTBT precipitated on the wall, and the blue GPC curve is for the dissolved fraction in the reaction flask. The dotted lines indicate the unimodal GPC curves for L-, M- and S-PCDTBT, respectively. Figure 3: GPC curves for split components and precipitated/dissolved fractions. ( a ) Polymer components (green, purple and red) extracted from the batch I sample. The dotted curves were virtually deconvoluted from the GPC data for the batch I sample. ( b ) The inset photograph shows the precipitated and dissolved products in a reaction flask after polymerization process. The red GPC curve is for the synthetic product of PCDTBT precipitated on the wall, and the blue GPC curve is for the dissolved fraction in the reaction flask. The dotted lines indicate the unimodal GPC curves for L-, M- and S-PCDTBT, respectively. Full size image Origin of the coexistence of three-component PCDTBTs We observed that the origin of the three-component coexistence was strongly related to the polymerization environment. For the PCDTBT polymerizations, toluene that has been widely adopted as a solvent to dissolve the starting materials was used in the reaction process. During the toluene-based polymerization with optimal conditions, we always encountered the formation of PCDTBT precipitate on the wall of the reaction flask (inset of Fig. 3b ). Notably, as shown in Fig. 3b , the GPC curves for the precipitated and dissolved portions largely agreed with L-PCDTBT, and the combination of M- and S-PCDTBT component curves, respectively. This observation has two important implications. First, toluene can either dissolve or precipitate the reaction product during the polymerization; the completely dissolved PCDTBT (that is, S- and M-PCDTBT) and marginally precipitated PCDTBT (that is, L-PCDTBT) can be separately or concurrently formed in the reaction flask. Second, the identical dissolving power of toluene solvent can lead that the dissolved and precipitated components are found at similar peak positions in every GPC data. Thus, it can be concluded that the low solubility of PCDTBT in toluene might lead to the occurrence of precipitation, and the precipitation (or the degree of precipitates) might itself divide synthetic environment or route, resulting in the multiple PCDTBT components during every synthesis. Characteristics of individual component PCDTBTs The chemically extracted component polymers exhibited quite different device characteristics. 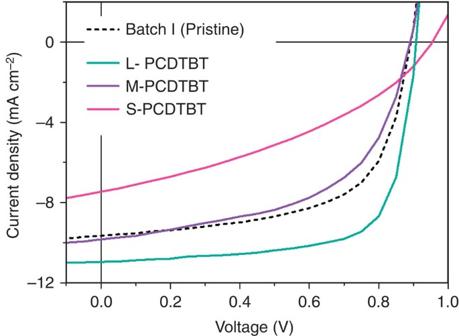Figure 4:J-Vcharacteristics for BHJ solar cells. J–Vcharacteristics for BHJ solar cells, respectively, with pristine batch I and its component PCDTBTs. Figure 4 shows the J–V characteristics of the PSC devices fabricated using the individual components: L-, M- and S-PCDTBT polymers. The detailed device parameters are summarized in Supplementary Table 1 . The L-PCDTBT-based PSC demonstrated a significantly enhanced efficiency (PCE≈7.04%) compared with that of the original pristine sample (batch I; PCE≈5.15%), whereas the S-PCDTBT-based device exhibited a poor efficiency (PCE≈2.62%). The M-PCDTBT component yielded a PCE similar to that of the pristine batch I sample. These results unambiguously support our earlier hypothesis that the unimodal distribution of high-MW polymers (here L-PCDTBT) would yield the best device performance and that the unwanted incorporation of lower-MW components (M- and S-PCDTBT) formed during the synthesis process causes the intrinsic properties of electronic polymers to deteriorate. Figure 4: J - V characteristics for BHJ solar cells. J–V characteristics for BHJ solar cells, respectively, with pristine batch I and its component PCDTBTs. Full size image To directly confirm our hypothesis, we intentionally added the S- and M-PCDTBT components into the L-PCDTBT component at various concentrations (that is, 5, 10, 20 and 50% by volume of solution). 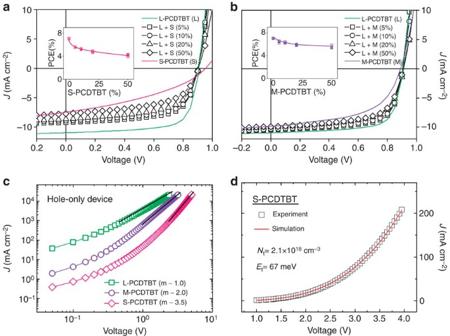Figure 5: Device performances on remixing and electrical characteristics of component PCDTBTs. (a) Variations in theJ–Vcharacteristics on the addition of S-PCDTBT to L-PCDTBT at various concentrations from 5 to 50%. (b) Variations in theJ–Vcharacteristics on the addition of M-PCDTBT to L-PCDTBT at various concentrations from 5 to 50%. The insets ina,bdepict the decreases in PCE that resulted from the addition of S- and M-PCDTBT to L-PCDTBT, respectively. (c) Log-log plot ofJ–Vdata for diode-type hole-only devices fabricated using the L-, M- and S-PCDTBT components as the active layers. The devices were constructed as follows: ITO\PEDOT:PSS\PCDTBT\MoOx\Ag. (d) ExperimentalJ–Vdata (empty squares) for the S-PCDTBT-based hole-only device and its simulated curve (solid red line). Figure 5a illustrates that the presence of the S-PCDTBT component had a considerable effect on the device performance. The device performance significantly decreased even with the incorporation of 5% S-PCDTBT into the L-PCDTBT component. Although the incorporation of the M-PCDTBT component also reduced the device performance ( Fig. 5b ), the effect was not as significant as in the case of S-PCDTBT. Therefore, we conclude that the low-MW S-PCDTBT component is the primary factor that is responsible for the variation in material quality in the PCDTBT system. This agrees well with the previous study of McGehee group, in which intentional contamination with monomers adversely affect the device performance [9] . Figure 5: Device performances on remixing and electrical characteristics of component PCDTBTs. ( a ) Variations in the J–V characteristics on the addition of S-PCDTBT to L-PCDTBT at various concentrations from 5 to 50%. ( b ) Variations in the J–V characteristics on the addition of M-PCDTBT to L-PCDTBT at various concentrations from 5 to 50%. The insets in a , b depict the decreases in PCE that resulted from the addition of S- and M-PCDTBT to L-PCDTBT, respectively. ( c ) Log-log plot of J–V data for diode-type hole-only devices fabricated using the L-, M- and S-PCDTBT components as the active layers. The devices were constructed as follows: ITO\PEDOT:PSS\PCDTBT\MoO x \Ag. ( d ) Experimental J–V data (empty squares) for the S-PCDTBT-based hole-only device and its simulated curve (solid red line). Full size image The substantial difference in material quality among the extracted components originates from the degree of trap density. When we estimated the trap density of the L-PCDTBT component by fabricating hole-only devices ( Supplementary Fig. 4a ), we found that the transport of holes in L-PCDTBT was governed by trap-free space-charge-limited conduction [18] . In contrast, the transport of holes in the S-PCDTBT component significantly deviated from the trap-free regime and exhibited typical trap-filling space-charge-limited conduction behavior ( Fig. 5c ) [19] . The trap density of S-PCDTBT was estimated to be approximately 2.1 × 10 18 cm −3 by fitting the measured data with a simple analytical equation ( Fig. 5d ) [20] , as explained in detail in the supporting information ( Supplementary Fig. 4b and Supplementary Table 2 ). Notably, the order of this trap density was quite high and close to the order of the effective density of HOMO states, which is typically assumed to be N HOMO ≈10 19 cm −3 (refs 20 , 21 ). Therefore, this analysis strongly supports our earlier hypothesis that the poor device performance of PCDTBT-based PSCs originates from the unintentional incorporation of trap-state-embedded moieties such as S-PCDTBT or/and M-PCDTBT. Effect of trap-embedded components on the burn-in loss In addition to adversely affecting the device efficiency through the inclusion of the trap-embedded moieties in S-PCDTBT, we discovered that this component has a more profound effect in PSCs. We measured the efficiency decay profiles ( Fig. 6a , Supplementary Fig. 5 and Supplementary Table 3 ) of the devices fabricated using these materials in a regular device structure. These devices were not encapsulated and were tested under an ambient atmosphere at T ≈25 °C and a relative humidity of ~50%. As a result of these tests, we found that the S-PCDTBT component is a possible origin for the ‘burn-in’ loss in PSCs. The devices fabricated using L-PCDTBT, which is believed to be completely absent of any of the trap-embedded moieties present in M- and S-PCDTBT, did not exhibit any significant ‘burn-in’ loss behavior during their initial operation; however, the inclusion of S-PCDTBT accelerated the early decrease in device performance to approach that observed for the pristine batch I. 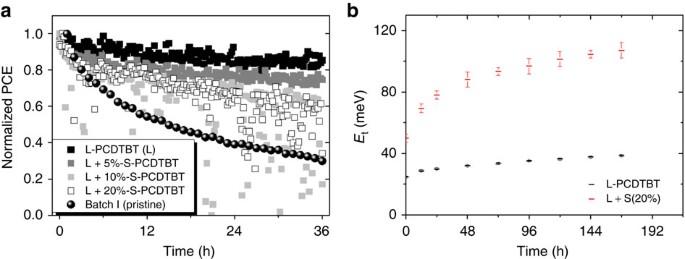Figure 6: Device degradation with embedding the S-fraction in the device. (a) Efficiency decay of the devices composed of pure L-PCDTBT and blends of L- and S-PCDTBT (5, 10 and 20%). The test devices were constructed using a regular device structure, and the tests were conducted at an ambient temperature of 25 °C and a relative humidity of 50% without encapsulation. (b) Characteristic width of exponential distribution of traps (Et) in PCDTBT:PC71BM hole-only devices. The hole-only devices were aged in air under one sun intensity with simulated AM1.5G solar spectrum. The evolutions ofEtwith aging time exhibited analogous manners to the degrading behaviours of the corresponding PCDTBT:PC71BM solar cells. Figure 6: Device degradation with embedding the S-fraction in the device. ( a ) Efficiency decay of the devices composed of pure L-PCDTBT and blends of L- and S-PCDTBT (5, 10 and 20%). The test devices were constructed using a regular device structure, and the tests were conducted at an ambient temperature of 25 °C and a relative humidity of 50% without encapsulation. ( b ) Characteristic width of exponential distribution of traps ( E t ) in PCDTBT:PC 71 BM hole-only devices. The hole-only devices were aged in air under one sun intensity with simulated AM1.5G solar spectrum. The evolutions of E t with aging time exhibited analogous manners to the degrading behaviours of the corresponding PCDTBT:PC 71 BM solar cells. Full size image For deeper understanding of their degradation behaviours, we probed the evolutions of photoinduced trap state formation, which has a strong correlation with the device degradation including burn-in loss [8] , [20] , [22] , and estimated the trap state distribution in energy [20] . First of all, to examine the photoinduced trap state formation, we fabricated hole-only devices (ITO\PEDOT:PSS\PCDTBT:PC 71 BM\MoO 3 \Ag), respectively, using L-PCDTBT and S-fraction-embedded PCDTBT as hole-transporting channels in the active BHJ layers. The devices were simply encapsulated with epoxy/glass, and stored in air under continuous light exposure of 1,000 W m −2 using a simulated AM1.5G spectrum, while the J–V characteristics of the devices were periodically measured in dark. As shown in Fig. 6b , the evolutions of the energetic breadths of trap distributions ( E t ) with respect to aging time were significantly different for the L-PCDTBT-based and S-fraction-embedded devices. The E t for the L-PCDTBT-based devices slightly widened from ~25 to ~35 meV over the initial course of aging (0 to 72 h), and after that period the trap width began to saturate. On the other hand, the E t for the S-fraction-embedded devices already exhibited a relatively broad span of ~50 meV, and significantly increased up to ~95 meV in the first 72 h of aging; even after that period, the E t value increased continuously with a gradual slope. For more intuitive perspective, when flipping the Fig. 6b upside down, one can apparently notice that the flipped curves exhibit very similar features to the decaying curves for the corresponding solar cells. Therefore, it is likely that the trap-width broadening is closely related to the device degradation, and the trap-embedded component such as S-PCDTBT promotes the trap-width broadening to accelerate the device degradation. In addition, the trap-width broadening could increase the possibility for the formation of deeper trap states in the bandgap because the E t determines the degree of deluged trap states into the bandgap from the valence band edge (that is, HOMO state) of the PCDTBT polymer [20] , [22] . By plotting the density of states as a function of energy ( E ) by equation (1): , where D t ( E ) is density of trap states, N t is the total trap states, E t is a characteristic width of trap distribution in energy, E HOMO is the transport state at valence band edge [20] , one can easily notice that the S-fraction-embedded device exhibits a deeply extended tail of trap-state distribution by ~500 meV in the bandgap after aging ( Supplementary Fig. 6a ). Because the Fermi levels ( E F ) of π -conjugated polymers with native defects (or natural doping) have been generally known to be in the range of a few hundred meV above the HOMO levels [22] , the tail reach of ~500 meV might be a significant value for the possibility of deeply trapped charges. The trapped charges that are lying deeper in the bandgap than the E F might proceed the photochemical reaction [8] , [22] , inducing charged defects to probably facilitate polymer oxidation. In contrast, for the L-PCDTBT-based device, the E t did not change much during the continuous light exposure, and the trap-distribution tail was slightly over the HOMO level (at best 100 meV; Supplementary Fig. 6b ). The narrow E t level and short tail-reach might suppress the photochemical chain reactions in the L-PCDTBT-based device. This argument is also further supported by the fact that the photoconductive signals of the transient photoconductivity decayed more slowly with an increase in the S-PCDTBT ratio in the photoactive layers ( Supplementary Fig. 7 and Supplementary Table 4 ) [23] , [24] . In addition to the photochemical reaction, structural defects or disorders also contribute to the trap-width broadening. As indicated by Beiley et al. [20] , in the PCDTBT films, the morphological change coincided with the broadening of energetic trap width. To examine the BHJ film stability, we thermally annealed the films of L-PCDTBT:PC 71 BM (1:4) and S-PCDTBT:PC 71 BM (1:4), and investigated their morphological changes using an atomic force microscopy. When the L-PCDTBT:PC 71 BM (1:4) BHJ film was thermally annealed at 150 °C for 1 h, there was no significant morphology change in the annealed film, as shown in atomic force microscopy image ( Supplementary Fig. 8a,b ). In contrast, the S-PCDTBT:PC 71 BM (1:4) BHJ film exhibited an apparent structural instability with several hundred nm-sized bumpy agglomerates arisen after the thermal annealing ( Supplementary Fig. 8c,d ). Consequently, we conclude that the trap-embedded moieties such as S-PCDTBT are likely to be not only the major source of deeper trap states, but also the potential cause for morphological instability of the BHJ films. Hence, the solar cells with trap-embedded moieties might degrade continuously even after burn-in. On the other hand, the elimination of trap-embedded moieties (for example, S-PCDTBT) mitigates the occurrence of deeper trap states and also enhances the morphological stability of the BHJ films, thereby suppressing the morphology changes and trap-width broadening during aging. Eventually, those effects might reduce the initial burn-in loss and suppress the decrease in the post-burn-in efficiency. Long-term stable polymer solar cells Finally, we fabricated inverted PSCs using the L-PCDTBT component with a device structure of ITO\ZnO\L-PCDTBT:PC 71 BM\MoO 3 \Ag to avoid the oxidation of the top metal electrode ( Supplementary Fig. 9a ). In this architecture, we obtained the highest value (PCE≈7.21%; Supplementary Fig. 9b ) ever reported in the PCDTBT system, which was much higher than that observed for any other pristine batch sample. To test long-term stability, we encapsulated an inverted device using the well-known epoxy-glass technique, as explained in the methods section. Then, we conducted a device-aging test under an ambient atmosphere at T ≈25 °C and a relative humidity of ~50%, and we recorded the J–V data every 30 min under continuous light exposure. The light source (LG sulphur plasma lamp, 6,000 K) was spectrally satisfied to the AM 1.5 G solar spectrum in the visible range. Under continuous light exposure using this lamp, we measured the device performance for 1,400 h. In contrast with the devices fabricated using the pristine batch I sample or the S-PCDTBT-containing sample, whose performance rapidly decayed ( Supplementary Fig. 10 ), the L-PCDTBT device survived for a considerably longer time; the device maintained more than 82% of its initial PCE even after 1,400 h, as shown in Fig. 7 . When we simulated the lifetime curve based on the regression tendency ( Supplementary Fig. 10 , Supplementary Table 5 ), it is noticed that a quite long lifetime can be expected in the PSCs with an extremely long lifetime expectancy over many years [8] , [25] . 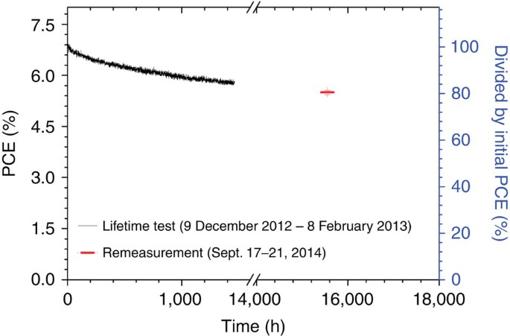Figure 7: Lifetime test. The solid line (black) indicates experimental data acquired during the lifetime test. The marker (red) represents the efficiencies remeasured ~2 years later using the exactly same device. It is notable that the device still survives despite ~2-year storage. Figure 7 additionally provides one more informative result. Despite ~2-year storage from the lifetime test, the device was still alive with little loss in efficiency. The remeasured J – V curves exhibit very similar characteristics to the last data measured at the end of the lifetime test 2 years ago ( Supplementary Fig. 11a ). Moreover, during the 5-day remeasurement, the J – V characteristics were unchanged; particularly, there was no loss in integrated photocurrent ( Supplementary Fig. 11b ). These results are somewhat unexpected and completely refutes the traditional view that polymer-based electronic devices cannot match the long-term stability of their inorganic counterparts. Although the remeasurement results are insufficient to justify the simulated prediction shown in Supplementary Fig. 10 , the data might be enough to confirm that the polymer solar cells are stronger than what we have predicted conventionally. For more precise lifetime prediction, more data obtained with much longer period should be supplemented with more precise simulation prediction. Figure 7: Lifetime test. The solid line (black) indicates experimental data acquired during the lifetime test. The marker (red) represents the efficiencies remeasured ~2 years later using the exactly same device. It is notable that the device still survives despite ~2-year storage. Full size image In this work, we selectively extracted the high-MW PCDTBT (that is, L-PCDTBT) by removing out the trap-embedded component PCDTBTs (that is, M- and S-PCDTBTs) from a pristine polymer batch based on the splits of unimodal MW distributions. The extracted resulting polymer, L-PCDTBT resulted in the significant enhancement of ~40% in PCE compared with that of the devices with the pristine PCDTBT. In addition, the elimination of the trap-embedded fractions significantly suppressed the photoactivated trap-width broadening and led to the almost absence of burn-in loss, suggesting a promising possibility of long-term stable PSCs. Moreover, during the study, we also noticed that a long-standing issue, so-called the ‘batch-to-batch’ variance could be originated from the random coexistence of the component PCDTBTs that might come separately from the precipitated and from the dissolved reaction products in the same reaction flask. Therefore, we expect that our findings might help to realize commercially viable PSCs satisfying their lifetime requirement. Materials PCDTBT was synthesized at both Gwangju Institute of Science and Technology (GIST) and Pusan National University (PNU) in South Korea using the same polymerization procedure ( Supplementary Fig. 2 ). PC 71 BM was purchased from Nano-C. All other commercial reagents, including solvents, which were used in this study were purchased from Aldrich and used as received. GPC measurement GPC measurements of the synthesized PCDTBT polymers were conducted by Professor Bazan’s group at center for polymers and organic solids of University of California, Santa Barbara (USCB). The PCDTBT polymers were difficult to characterize using normal room-temperature GPC with chloroform as the solvent because of their poor solubilities. To completely dissolve the polymer samples, we used high-temperature GPC at 150 °C with an injected concentration of C inj ~0.5 mg ml −1 using the highly soluble and high-boiling point solvent 1,2,4-trichlorobenzene. The columns were also calibrated using the EasiCalw PS-1 standard (PL) and several individual narrow PS standards (Polyscience Inc. and PL) with C inj =0.25–0.5 mg ml −1 (depending on MW). All sample solutions, including both the PS standards and the PCDTBT solutions, were filtered using a 2-μm frit after the samples were dissolved in 1,2,4-trichlorobenzene at 150 °C overnight. Device fabrication BHJ solar cells were fabricated as follows: first, ITO-sputtered glass substrates were cleaned using a detergent solution and then ultrasonicated in deionized water, acetone and isopropyl alcohol step by step. After the cleaning process, the substrates were dried overnight in a drying oven at 80 °C. Then, the dried ITO substrates were transferred into a ultraviolet–ozone cleaner. After the ultraviolet–ozone treatment, a hole-transport layer (HTL) of PEDOT:PSS (AI 4083, as purchased) was spin cast onto the cleaned ITO substrates and dried under ambient air. The HTL-coated substrates were transferred into an N 2 -filled glove box for the formation of the photoactive layers. The photoactive layers were spin cast using BHJ solutions that consisted of PCDTBT (5 mg ml −1 in DCB) and PC 71 BM (20 mg ml −1 in DCB). The BHJ films were dried at 60 °C for 30 min to vaporize the solvent remaining in the films. An electron-transport layer of TiO x (~10 nm) was formed on the photoactive layers by spin casting a diluted TiO x precursor solution. To deposit the top metal electrode, the samples were transferred into a vacuum chamber and aluminium (Al) was then thermally evaporated onto the samples at <10 −7 Torr. The overall device structure was glass\ITO\PEDOT:PSS\PCDTBT:PC 71 BM\TiO x \Al. For the inverted device structure (glass\ITO\ZnO\PCDTBT:PC 71 BM\MoO 3 \Ag), ZnO was introduced as an electron-transport layer (~20 nm) by spin casting a ZnO precursor sol (Zn acetate dissolved in IPA) onto a clean ITO glass substrate. The active layers were deposited using the same procedure as that used to fabricate the regular device. MoO 3 was evaporated onto the active layer in the vacuum chamber (<10 −7 Torr) as an HTL (~10 nm) for both the inverted device and the hole-only device (glass\ITO\PEDOT:PSS\PCDTBT\MoO 3 \Ag). For the long-term reliability tests, the devices were encapsulated within glass slides of ~1 mm in thickness using a two-part epoxy resin (Loctite Instant Mix 5 Minute Epoxy). Device measurement Current–density–voltage ( J–V ) characteristics were measured using a Keithley 236 Source Measure Unit for the hole-only devices and PSCs in the dark and/or under illumination (100 mW cm −2 , AM 1.5 G) in an N 2 -filled glove box. The active area was defined by the area of the top metal electrode (4.64 mm 2 ). The EQEs were measured using a PV Measurement IPCE system (PV Measurements, Inc.). Reliability test An LG sulphur plasma lamp (6,000 K) was used as the illumination source for the lifetime test. Except in the ultraviolet range, the lamp provided a decent spectral match to the AM 1.5 solar spectrum in the visible region. The test chamber was maintained at a temperature of 25±2 °C and a relative humidity of ~50%, and the test devices were periodically monitored under continuous illumination for a given duration for each test. How to cite this article: Kong, J. et al. Long-term stable polymer solar cells with significantly reduced burn-in loss. Nat. Commun. 5:5688 doi: 10.1038/ncomms6688 (2014).